Aquaporin-3-mediated hydrogen peroxide transport is required for NF-κB signalling in keratinocytes and development of psoriasis Aquaporin 3 (AQP3), a water/glycerol channel protein, has been found to transport hydrogen peroxide (H 2 O 2 ). Here, we show that H 2 O 2, imported via AQP3, is involved in nuclear factor-κB (NF-κB) signalling in keratinocytes and in the pathogenesis of psoriasis. IL-23-mediated induction of psoriasis is reduced in AQP3 knockout mice (AQP3 −/− ), and is accompanied by impaired NF-κB activation and intracellular H 2 O 2 accumulation. In primary keratinocyte cultures, cellular import of H 2 O 2 produced by membrane NADPH oxidase 2 (Nox2) in response to TNF-α is facilitated by AQP3 and required for NF-κB activation by regulation of protein phosphatase 2A. As AQP3 associates with Nox2, we propose that this interplay constitutes H 2 O 2 -mediated signalling in response to TNF-α stimulation. Collectively, these data indicate that AQP3-facilitated H 2 O 2 transport is required for NF-κB activation in keratinocytes in the development of psoriasis. Psoriasis is a chronic inflammatory skin disease characterized by raised plaques, epidermal hyperplasia and infiltration of leukocytes into the skin, though its precise pathogenesis mechanism remains unclear [1] , [2] . Recent genetic studies have advanced our understanding of the pathogenesis of psoriasis. Ten genome-wide association studies have identified more than 20 susceptible loci in psoriasis and suggested several pathogenesis mechanisms, including skin barrier functions, IL-17 and IL-23 signalling, TNF-α and NF-κB signalling and HLA-C [3] , [4] , [5] . IL-23 and TNF-α-targeted therapies, which neutralize subunits of cytokines IL-12/23 or TNF-α respectively, are in clinical use and improve the quality of life for psoriasis patients [6] . A recent clinical report showed that an IL-17A neutralizing monoclonal antibody also had efficacy in psoriasis [7] , [8] . There have also been recent advances in signalling pathways involved in the pathogenesis of psoriasis. Increasing evidence implicates IL-17 as a centrally important cytokine in psoriatic skin, which stimulates keratinocytes and promotes chronic inflammation [3] . There is also recent evidence that activation of NF-κB signalling exacerbates psoriatic lesions, potentially by induction of various genes for cytokines, chemokines and growth factors [1] , [9] , [10] . However, the underlying mechanisms of how these pathways produce psoriasis remain unresolved. Aquaporin-3 (AQP3), a member of the aquaporin water channel family, is a water- and glycerol-transporting protein that is involved in various cellular functions including cell proliferation and migration [11] . Previous studies have shown the involvement of AQP3 expression in skin diseases, including wound healing, tumorigenesis and atopic dermatitis, in which their pathogenesis was attributed to the AQP3 water or glycerol transport function in epidermal keratinocytes [12] , [13] , [14] . Building on a study reporting AQP3-facilitated cellular uptake of H 2 O 2 (ref. 15 ), a reactive oxygen species (ROS), we reported the involvement of AQP3-mediated H 2 O 2 in T-cell signalling in cutaneous contact hypersensitivity [16] . We showed that extracellular H 2 O 2 produced in response to CXCL12 stimulation was transported into T cells by AQP3, which facilitated CXCL12-dependent cell signalling and T cell migration. Because H 2 O 2 is emerging as an important second messenger in cell signalling [17] , [18] , we postulated that AQP3-facilitated intracellular H 2 O 2 might be implicated in a variety of human disease, including the focus of the study here, psoriasis. We report here that AQP3 is required for TNF-α-induced NF-κB activation in keratinocytes and the development of psoriasis by a mechanism involving TNF-α-induced generation of extracellular H 2 O 2 followed by its intracellular transport by AQP3. An in vivo mouse model of psoriasis showed remarkably reduced pathology in an AQP3-deficient background, in which continuous NF-κB activation and a higher H 2 O 2 level in epidermal keratinocytes were suppressed by AQP3 deficiency. Reduced IL-23-induced psoriasis-like inflammation in AQP3 −/− mice Although previous reports showed reduced AQP3 staining or an altered pattern of AQP3 distribution in psoriatic skin, microarray and RNA-seq studies have suggested an upregulation of AQP3 expression [19] , [20] , [21] , [22] . AQP3 immunostaining was done on 18 human psoriatic skin samples. We found strong AQP3 immunostaining, with two patterns of AQP3 localization in keratinocytes: typical plasma membrane staining for eight specimens, and mixed plasma membrane/cytoplasmic staining for nine specimens ( Fig. 1a , left, insert). One specimen showed weak AQP3 staining. Immunofluorescence showed AQP3 expression in CD3 + T cells infiltrating in the dermis ( Fig. 1a , right). AQP3 transcript expression was more than eight-fold greater in keratinocytes than in CD3 + T cells by PCR with reverse transcription (RT–PCR; Supplementary Fig. 1a ). 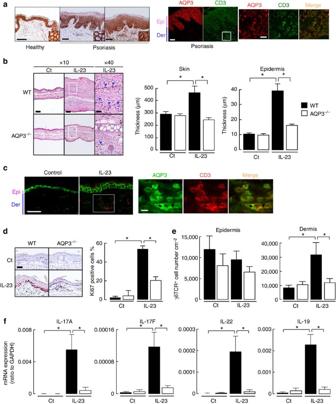Figure 1: Impaired IL-23-induced psoriasis-like skin in AQP3−/−mice. (a) Left: representative immunohistochemical staining for AQP3 in the skin from five healthy volunteers and 18 psoriatic patients. Right: immunostaining with anti-AQP3 (cy3, red) and anti-CD3 (FITC, green) in psoriatic skin. Scale bar, 100 μm. Epi, epidermis; der, dermis. (b–f) IL-23 (500 ng) or vehicle control (PBS) was intradermally injected daily into the ear skin of WT and AQP3−/−mice for 4 days. Skin samples were excised at 24 h after the final IL-23 injection. (b) Left: haematoxylin and eosin staining of ears from WT and AQP3−/−mice. Scale bar, 100 μm. Arrow head, infiltrating lymphocytes. Right: whole skin and epidermal thickness determined from haematoxylin and eosin staining (s.e.,n=5, *P<0.01 byt-test).(c) Immunostaining with anti-AQP3 (FITC, green) and anti-CD3 (cy3, red) in WT mouse skin. Scale bar, 100 μm (left), 20 μm (right). (d) Left: representative immunohistochemical staining for Ki67. Right: the ratio of Ki67 positive cells in the epidermis (s.e.,n=3, *P<0.01 byt-test). (e) CD3+γδTCR+cell numbers in epidermis and dermis from WT and AQP3−/−mice analysed by flow cytometry (s.e.,n=4–5, *P<0.01 byt-test). (f) mRNA expression of IL-17A, IL-17F, IL-22 and IL-19 in skin tissues determined by real-time RT–PCR (s.e.,n=4–5,*P<0.01 byt-test). Data are expressed as the ratio to GAPDH. Figure 1: Impaired IL-23-induced psoriasis-like skin in AQP3 −/− mice. ( a ) Left: representative immunohistochemical staining for AQP3 in the skin from five healthy volunteers and 18 psoriatic patients. Right: immunostaining with anti-AQP3 (cy3, red) and anti-CD3 (FITC, green) in psoriatic skin. Scale bar, 100 μm. Epi, epidermis; der, dermis. ( b – f ) IL-23 (500 ng) or vehicle control (PBS) was intradermally injected daily into the ear skin of WT and AQP3 −/− mice for 4 days. Skin samples were excised at 24 h after the final IL-23 injection. ( b ) Left: haematoxylin and eosin staining of ears from WT and AQP3 −/− mice. Scale bar, 100 μm. Arrow head, infiltrating lymphocytes. Right: whole skin and epidermal thickness determined from haematoxylin and eosin staining (s.e., n =5, * P <0.01 by t -test). ( c ) Immunostaining with anti-AQP3 (FITC, green) and anti-CD3 (cy3, red) in WT mouse skin. Scale bar, 100 μm (left), 20 μm (right). ( d ) Left: representative immunohistochemical staining for Ki67. Right: the ratio of Ki67 positive cells in the epidermis (s.e., n =3, * P <0.01 by t -test). ( e ) CD3 + γδTCR + cell numbers in epidermis and dermis from WT and AQP3 −/− mice analysed by flow cytometry (s.e., n =4–5, * P <0.01 by t -test). ( f ) mRNA expression of IL-17A, IL-17F, IL-22 and IL-19 in skin tissues determined by real-time RT–PCR (s.e., n =4–5,* P <0.01 by t -test). Data are expressed as the ratio to GAPDH. Full size image We used an experimental mouse model of IL-23-induced psoriasis to study the potential role of AQP3 in the pathogenesis of psoriasis [23] , [24] . IL-23 was injected into the skin of the ear of wild-type (WT) and AQP3 knockout (AQP3 −/− ) mice. Consistent with previous reports, injection of IL-23 into WT skin induced marked ear swelling, accompanied by pronounced acanthosis, hyperparakeratosis and lymphocytic infiltration ( Fig. 1b , left). The skin of AQP3 −/− mice showed remarkably less swelling and inflammation after injection of IL-23. Whole skin and epidermal thickness in haematoxylin and eosin-stained sections showed significantly reduced swelling and hyperkeratosis in AQP3 −/− mice ( Fig. 1b , right). Immunostaining showed AQP3 expression in keratinocytes and dermal CD3 + T cells in the psoriasis-induced mouse skin ( Fig. 1c ), similar to observations in human psoriatic skin. The AQP3 messenger RNA (mRNA) expression level in isolated epidermal cells was similar in control and IL-23-treated WT skin ( Supplementary Fig. 1b ). Immunoblot analysis showed that the increased AQP3 expression after IL-23 injection was associated with greater keratin 5 and 14 expression in epidermis compared with control skin ( Supplementary Fig. 1c ). Immunohistochemical analysis showed that IL-23 application remarkably increased Ki67 + keratinocytes in WT but not in AQP3 −/− epidermis, suggesting that IL-23 stimulation induced keratinocytes proliferation in WT skin ( Fig. 1d ). These data indicate that the higher AQP3 expression by immunoblotting is due to an increase in proliferative keratinocytes. Previous studies showed that IL-23 injection increased the number of CD3 + γδTCR + cells (γδ T cells) in the dermis, which contributes to the development of psoriatic skin by IL-17 production [25] . We confirmed that CD3 + γδTCR + cells specifically accumulated in IL-23-treated WT skin ( Supplementary Fig. 1d ). Fluorescence-activated cell sorting (FACS) analysis showed greater numbers of γδ T cells in the dermis after IL-23 treatment in WT than in AQP3 −/− mice ( Fig. 1e ). Quantitative RT–PCR analysis revealed that continuous IL-23 injection increased mRNAs encoding IL-17A, IL-17F, IL-22 and IL-19 in WT epidermis, as previously reported, with reduced elevations in AQP3 −/− epidermis ( Fig. 1f ). These data indicate the involvement of AQP3 in the development of psoriasis in the IL-23 mouse model. Impaired psoriasis is dependent on AQP3 expression Previous studies implicated a critical role for both T cells and keratinocytes in the pathogenesis of psoriasis as well as in the psoriatic mouse model induced by IL-23 application [2] , [3] , [23] , [24] , [25] . AQP3 was found to be expressed in epidermal keratinocytes and T cells in psoriatic skin ( Fig. 1a,c ). To investigate the potential significance of AQP3 expression in these cell types individually, lethally irradiated WT and AQP3 −/− mice (recipients) were reconstituted with bone marrow (BM) cells from WT and AQP3 −/− mice (donors; Supplementary Fig. 2a ). When these mice were injected with IL-23 to induce psoriatic skin changes, ear swelling measured with a micrometer was increased in chimeric mice produced by transferring WT BM cells into WT recipients ( Fig. 2a,b ). In contrast, chimeric mice produced by transferring WT BM cells into AQP3 −/− recipients showed reduced IL-23-induced ear swelling, indicating that the development of psoriasis requires the expression of AQP3 in keratinocytes. Transfer of AQP3 −/− BM into WT recipients also suppressed IL-23-induced ear swelling, suggesting the involvement of AQP3 expression in haematopoietic cells, probably in T cells ( Fig. 2a,b ). 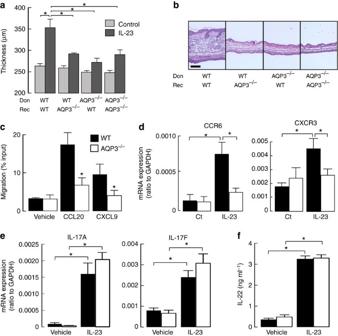Figure 2: Impaired IL-23-induced psoriasis is dependent on AQP3 expression in both keratinocytes and T cells. (a,b) IL-23-induced psoriatic model using bone marrow (BM) cell-transferred mice. Recipient WT and AQP3−/−mice (Rec) received transplants of BM cells from donor WT and AQP3−/−mice (Don). (a) Ear thickness at 24 h after final injections (s.e.,n=5, *P<0.01 byt-test). (b) Representative haematoxylin and eosin staining. Scale bar, 100 μm. (c) Chemotaxis assay. The migration efficiency of CD3+T cells toward the ligands CCL20 (100 ng ml−1) or CXCL9 (100 ng ml−1) was determined using a transwell chamber with 5 μm pores. Data are expressed as the percentage of applied cells (s.e.,n=5, *P<0.01 byt-test). (d) mRNA expression levels of CCR6 in epidermis (left) and CXCR3 in dermis (right) by real-time RT–PCR (s.e.,n=5, *P<0.01 byt-test). (e) mRNA expression levels of IL-17A and IL-17F by real-time RT–PCR in sorted T cells incubated with IL-23 in the presence of CD3/28 for 3 days (s.e.,n=5, *P<0.01 byt-test). Data are expressed as the IL-17/GAPDH ratio. (f) IL-22 level by ELISA in the culture medium with IL-23 in the presence of anti-IL-4 and anti-IFNγ for 3 days (s.e.,n=5, *P<0.01 byt-test). Figure 2: Impaired IL-23-induced psoriasis is dependent on AQP3 expression in both keratinocytes and T cells. ( a , b ) IL-23-induced psoriatic model using bone marrow (BM) cell-transferred mice. Recipient WT and AQP3 −/− mice (Rec) received transplants of BM cells from donor WT and AQP3 −/− mice (Don). ( a ) Ear thickness at 24 h after final injections (s.e., n =5, * P <0.01 by t -test). ( b ) Representative haematoxylin and eosin staining. Scale bar, 100 μm. ( c ) Chemotaxis assay. The migration efficiency of CD3 + T cells toward the ligands CCL20 (100 ng ml −1 ) or CXCL9 (100 ng ml −1 ) was determined using a transwell chamber with 5 μm pores. Data are expressed as the percentage of applied cells (s.e., n =5, * P <0.01 by t -test). ( d ) mRNA expression levels of CCR6 in epidermis (left) and CXCR3 in dermis (right) by real-time RT–PCR (s.e., n =5, * P <0.01 by t -test). ( e ) mRNA expression levels of IL-17A and IL-17F by real-time RT–PCR in sorted T cells incubated with IL-23 in the presence of CD3/28 for 3 days (s.e., n =5, * P <0.01 by t -test). Data are expressed as the IL-17/GAPDH ratio. ( f ) IL-22 level by ELISA in the culture medium with IL-23 in the presence of anti-IL-4 and anti-IFNγ for 3 days (s.e., n =5, * P <0.01 by t -test). Full size image We next determined the contribution of AQP3-facilitated T-cell chemotaxis to the development of psoriasis, based on our recent demonstration that AQP3 is required for T-cell chemotaxis [16] . The mRNA levels of CCL20, CXCL9 and CXCL10, key chemokines to recruit T cells or dendritic cells during the development of psoriasis [26] , were remarkably increased in IL-23-treated WT skin ( Supplementary Fig. 2b ). The chemotaxis of CD3 + T cells to CCL20 or CXCL9 was significantly reduced in AQP3 −/− cells ( Fig. 2c ). We also found that expression of CCR6 and CXCR3, the receptors of CCL20 and CXCL9 respectively, was decreased in IL-23-treated AQP3 −/− skin compared with WT skin ( Fig. 2d ). These results suggest that the impaired T-cell chemotaxis leads to less accumulation of CCR6 + and CXCR3 + T cells in AQP3 −/− skin. During the development of psoriasis induced by IL-23 application, IL-17 and IL-22 production by T cells in response to IL-23 stimulation is crucial for the following steps [23] , [24] , [25] . We found comparable expression of mRNA encoding IL-17A/F in WT and AQP3 −/− primary cultured T cells, as well as comparable IL-22 production ( Fig. 2e,f ). FACS analysis also showed a comparable ratio of IL-17 expressing cells among γδT cells in skin-draining lymph nodes in WT and AQP3 −/− mice following IL-23 application ( Supplementary Fig. 2c ). From these results, we propose that AQP3 deficiency results in the impaired T-cell migration into the dermal and epidermal layers, which reduces downstream immune response during the development of psoriasis. AQP3 deficiency suppresses NF-κB activation and H 2 O 2 induction We next sought to elucidate the role of AQP3 in keratinocytes in the pathogenesis of psoriasis, since the reduced psoriasis in AQP3 −/− mice cannot be accounted for by functions of AQP3 reported previously [13] , [14] . Several studies suggest an important role of NF-κB in the pathogenesis of psoriasis [1] , [9] , [10] , including overexpression of active phosphorylated NF-κB in psoriatic epidermis [27] , [28] . Immunostaining showed a much greater number of positive keratinocytes for phospho-p65 and phospho-IKKα/β in IL-23-treated WT skin than control skin, as found in humans [27] , [28] ( Fig. 3a , Supplementary Fig. 3a ). AQP3 −/− epidermis showed fewer cells positive for phospho-p65 and phospho-IKKα/β compared with WT skin. Immunoblot also showed reduced IL-23-induced phosphorylation of Iκβα and its degradation in AQP3 −/− epidermis ( Fig. 3b , Supplementary Fig. 7 ), indicating that NF-κB was activated by IL-23 application in WT but not in AQP3 −/− skin. 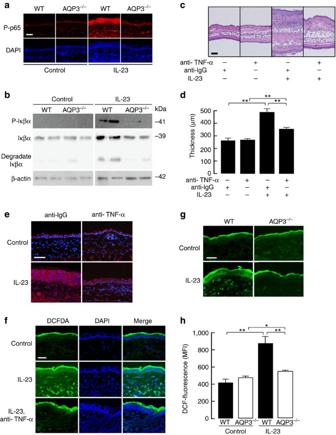Figure 3: AQP3 deficiency impairs H2O2elevation and NF-κB activation in IL-23-treated skin. (a,b) Mice were injected with IL-23 into the ear as described inFig. 1. (a) Immunostaining of phospho-p65 in PBS (control) or IL-23 injected WT and AQP3−/−skin. Scale bar, 100 μm. (b) Representative immunoblot analysis using antibodies against phospho-Iκβα, Iκβα and β-actin. Experiments were performed in two other independent experiments with similar results. (c–e) Haematoxylin and eosin staining (c), ear thickness (d) and phospho-p65 immunostaining (e) of ears from WT mice treated daily with IL-23 or PBS (control) in the presence of anti-TNF-α blocking monoclonal antibody or isotype control. (f) H2DCFDA fluorescence in the skin treated with IL-23 (three continuous applications) with or without anti-TNF-α antibody. Anti-TNF-α antibody was injected 1 h before sampling. (g) H2DCFDA fluorescence in WT and AQP3−/−skin treated daily with PBS (control) or IL-23 by fluorescence microscopy. (h) The mean fluorescence intensity (MFI) of H2DCFDA by FACS analysis in epidermal cells (s.e.,n=5, *P<0.05, **P<0.01 byt-test). Figure 3: AQP3 deficiency impairs H 2 O 2 elevation and NF-κB activation in IL-23-treated skin. ( a , b ) Mice were injected with IL-23 into the ear as described in Fig. 1 . ( a ) Immunostaining of phospho-p65 in PBS (control) or IL-23 injected WT and AQP3 −/− skin. Scale bar, 100 μm. ( b ) Representative immunoblot analysis using antibodies against phospho-Iκβα, Iκβα and β-actin. Experiments were performed in two other independent experiments with similar results. ( c – e ) Haematoxylin and eosin staining ( c ), ear thickness ( d ) and phospho-p65 immunostaining ( e ) of ears from WT mice treated daily with IL-23 or PBS (control) in the presence of anti-TNF-α blocking monoclonal antibody or isotype control. ( f ) H 2 DCFDA fluorescence in the skin treated with IL-23 (three continuous applications) with or without anti-TNF-α antibody. Anti-TNF-α antibody was injected 1 h before sampling. ( g ) H 2 DCFDA fluorescence in WT and AQP3 −/− skin treated daily with PBS (control) or IL-23 by fluorescence microscopy. ( h ) The mean fluorescence intensity (MFI) of H 2 DCFDA by FACS analysis in epidermal cells (s.e., n =5, * P <0.05, ** P <0.01 by t -test). Full size image Reported evidence suggests that TNF-α-dependent NF-κB signalling is required for the development of psoriasis [1] , [9] , [10] . A previous study suggested that IL-23-induced psoriatic changes are dependent on TNF-α-mediated cell signalling in mice, as pretreatment with a blocking monoclonal TNF-α antibody reduced psoriatic changes in 129SvEv mice [24] . We confirmed that administration of TNF-α antibody attenuated IL-23-induced skin swelling in WT mice (C57B/6 background; Fig. 3c,d ). NF-κB activation was suppressed with TNF-α antibody, with significantly fewer phospho-p65-positive cells than with an IgG-isotype control ( Fig. 3e , Supplementary Fig. 3c ), which is consistent with the data in human psoriasis [27] . It has been also suggested that TNF-α-dependent NF-κB activation is H 2 O 2 -regulated [29] , [30] . To test our hypothesis that AQP3-mediated intracellular H 2 O 2 is a central signalling event in the development of psoriasis, we measured cellular H 2 O 2 levels in skin using a previously described method [31] . Injections of IL-23 increased intracellular H 2 O 2 in epidermal keratinocytes and in some dermal cells in WT mice ( Fig. 3f ). The administration of TNF-α antibody before IL-23 application reduced the increase in intracellular in H 2 O 2 ( Fig. 3f ), suggesting IL-23-induced H 2 O 2 accumulation was partially dependent on TNF-α cell signalling. In addition, the H 2 O 2 level was greater in WT epidermal cells than in AQP3 −/− cells after IL-23 application ( Fig. 3g ). Finally, we quantified cellular H 2 O 2 in epidermal cells by FACS analysis. After trypsinization of the epidermal sheet, single-cell suspensions were incubated with H 2 DCFDA, as validated for measurement of intracellular H 2 O 2 ( Supplementary Fig. 3d ). The H 2 DCFDA fluorescence in epidermal cells showed significantly higher H 2 O 2 in WT than in AQP3 −/− epidermal cells after IL-23 application ( Fig. 3h ). As further evidence for the involvement of AQP3 in the development of psoriasis, we performed an imiquimod (IMQ)-induced psoriasis model [32] . The IMQ-treated AQP3 −/− mice showed reduced ear swelling and psoriasis-like phenotype (acanthosis and lymphocytic infiltration) compared with WT skin ( Supplementary Fig. 4a,b ). AQP3 was expressed in a wide range of hyperplastic psoriatic epidermis ( Supplementary Fig. 4c ). The IMQ-treated WT epidermal cells showed an increased number of phospho-p65-positive and a higher ROS level, as seen in IL-23-treated WT skin ( Supplementary Fig. 4d,e ). Together, these findings provide evidence for involvement of AQP3 in H 2 O 2 induction and NF-κB activation in IL-23-induced psoriatic changes in skin, which are dependent on TNF-α signalling. Impaired TNF-α-induced NF-κB activation in AQP3 −/− We next investigated the involvement of AQP3 in TNF-α-induced NF-κB activation in primary keratinocytes from WT and AQP3 −/− mice. Immunoblot analysis showed that 1-h TNF-α stimulation induced the phosphorylation of p65/NF-κB in WT cells, which was reduced in AQP3 −/− cells ( Fig. 4a , Supplementary Fig. 6a and 7 ). TNF-α-induced signalling is mediated by one of the two cell-surface receptors, TNFR1 and TNFR2 (ref. 33 ). Classical NF-κB activation following TNF-α stimulation is initiated by recruitment of the death domain-containing proteins RIP1 and TRADD, after binding of TNF receptor (TNFR)-associated factor 2 (TRAF2) to TNFR1 (refs 33 , 34 ). A previous study showed that the recruitment of TRAF2 to TNFR1 in response to TNF-α was dependent on the ROS level [35] . Immunoprecipitation with anti-TNFR1 showed that AQP3 deficiency did not affect the recruitment of TRAF2 and RIP1 to TNFR1 upon TNF-α stimulation ( Fig. 4b , Supplementary Fig. 7 ). In contrast, AQP3 −/− keratinocytes showed reduced TNF-α-induced phosphorylation of IKKβ and Iκβα and degradation of Iκβα ( Fig. 4a , Supplementary Figs 6a and 7 ). 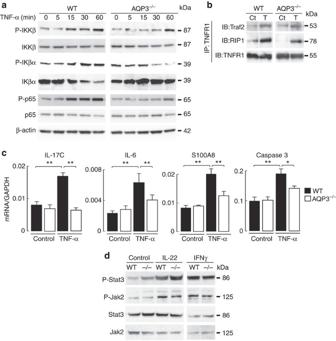Figure 4: Impaired TNF-α-induced NF-κB activation in AQP3-deficient keratinocytes. (a,b) Primary keratinocytes from WT and AQP3−/−mice were incubated with TNF-α (100 ng ml−1) for 5 min to 1 h. (a) Representative immunoblot using antibodies against phospho-IKKβ, IKKβ, phospho-Iκβα, Iκβα, phospho-p65, p65 and β-actin at indicated times. (b) Cell lysate (TNF-α, 100 ng ml−1, 5 min) was immunoprecipitated with anti-TNFR1. Immunoblot was performed with anti-Traf2, anti-RIP1 and anti-TNFR1. Ct, control; T, TNF-α. Experiments inaandbwere performed in two other independent experiments with similar results. (c) mRNA expression in primary keratinocytes by real-time RT–PCR. Cells from WT and AQP3−/−mice were incubated with TNF-α (100 ng ml−1) for 24 h. Data are expressed as the ratio to GAPDH (s.e.,n=5, *P<0.05, **P<0.01 byt-test). (d) Primary keratinocytes from WT and AQP3−/−mice were incubated with IL-22 (100 ng ml−1, 10 min) or IFNγ (100 ng ml−1, 10 min). Representative immunoblot analysis with anti-phospho-Stat3, -Jak2, Stat3 or Jak2. A second set of experiments gave similar results. Figure 4: Impaired TNF-α-induced NF-κB activation in AQP3-deficient keratinocytes. ( a , b ) Primary keratinocytes from WT and AQP3 −/− mice were incubated with TNF-α (100 ng ml −1 ) for 5 min to 1 h. ( a ) Representative immunoblot using antibodies against phospho-IKKβ, IKKβ, phospho-Iκβα, Iκβα, phospho-p65, p65 and β-actin at indicated times. ( b ) Cell lysate (TNF-α, 100 ng ml −1 , 5 min) was immunoprecipitated with anti-TNFR1. Immunoblot was performed with anti-Traf2, anti-RIP1 and anti-TNFR1. Ct, control; T, TNF-α. Experiments in a and b were performed in two other independent experiments with similar results. ( c ) mRNA expression in primary keratinocytes by real-time RT–PCR. Cells from WT and AQP3 −/− mice were incubated with TNF-α (100 ng ml −1 ) for 24 h. Data are expressed as the ratio to GAPDH (s.e., n =5, * P <0.05, ** P <0.01 by t -test). ( d ) Primary keratinocytes from WT and AQP3 −/− mice were incubated with IL-22 (100 ng ml −1 , 10 min) or IFNγ (100 ng ml −1 , 10 min). Representative immunoblot analysis with anti-phospho-Stat3, -Jak2, Stat3 or Jak2. A second set of experiments gave similar results. Full size image TNF-α-dependent NF-κB signalling regulates inflammation and apoptosis during the development of psoriasis [36] . Quantitative RT–PCR of primary keratinocytes showed that TNF-α stimulation increased levels of IL-17c, IL-6 and S100A8, which are related to inflammation in response to NF-κB activation, with lesser increases in AQP3 −/− keratinocytes ( Fig. 4c ). AQP3 deficiency also attenuated the increase in the response to TNF-α of caspase 3, a key enzyme in the apoptotic pathway. To verify the specific role of AQP3 in NF-κB signalling, we examined Jak2/Stat3 activation in response to IL-22 or interferon gamma (INFγ), which are also thought to be key cell signalling molecules in the development of psoriasis [37] , [38] . We found comparable phosphorylation of Jak2 and Stat3 with IL-22 or INFγ stimulation ( Fig. 4d , Supplementary Fig. 7 ). These results suggest that AQP3 expression in keratinocytes is required for NF-κB activation in response to TNF-α stimulation. TNF-α-mediated increase in intracellular H 2 O 2 depends on AQP3 There is increasing evidence that H 2 O 2 plays an important role in the regulation of NF-κB [29] , [30] , [39] . We hypothesized that AQP3-facilitated intracellular H 2 O 2 accumulation is involved in NF-κB activation in the presence of TNF-α. First, we investigated whether AQP3 can transport extracellular H 2 O 2 into keratinocytes. Intracellular H 2 O 2 was measured in primary keratinocyte cultures from WT and AQP3 −/− mice after extracellular addition of 10–300 μM H 2 O 2 using the fluorescent dye CM-H 2 DCFDA, which reacts with ROS including H 2 O 2 . We found that cellular H 2 O 2 increased to a significantly greater extent in WT than in AQP3 −/− keratinocytes, demonstrating the involvement of AQP3 in H 2 O 2 transport in keratinocytes ( Fig. 5a,b ). Cell morphology and apoptosis after incubation with H 2 O 2 was comparable in WT and AQP3 −/− cells ( Supplementary Fig. 5a,b ). 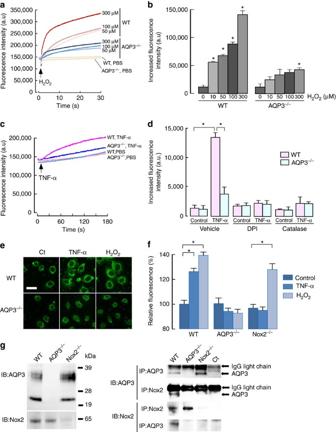Figure 5: AQP3-dependent H2O2permeability in keratinocytes. (a,b) H2O2uptake into primary cultured keratinocytes. Keratinocytes were incubated with H2O2(10 to 300 μM), and cellular H2O2was detected using CM-H2DCFDA fluorescence using a plate reader. (a) Representative fluorescence intensity of CM-H2DCFDA. (b) Increased fluorescence intensity at 15 s after addition of H2O2(s.e.,n=5, *P<0.01, H2O2added versus control cells byt-test). (c–d) Intracellular H2O2was monitored by CM-H2DCFDA fluorescence with TNF-α stimulation (100 ng ml−1). (c) Representative fluorescence intensity in WT and AQP3−/−cells. (d) Cells were incubated with DPI (5 μM), catalase (2,000 U ml−1) or vehicle (PBS) for 30 min, and followed by TNF-α (100 ng ml−1) for 30 s (s.e.,n=5, *P<0.01 byt-test). (e) WT and AQP3−/−cells transfected with HyPer were incubated with TNF-α (100 ng ml−1) or H2O2(100 μM) for 3 min. Representative immunofluorescence. Scale bar, 20 μm. (f) Cellular H2O2after stimulation by TNF-α (100 ng ml−1) or H2O2(100 μM) in primary keratinocytes from WT, AQP3−/−, or Nox2−/−mice using CM-H2DCFDA fluorescence (1 min, s.e.,n=7, *P<0.01 byt-test). (g) Left: immunoblot of AQP3 and Nox2 in membrane-rich fraction from WT, AQP3−/−and Nox2−/−keratinocytes. Right: cell lysates by RIPA were immunoprecipitated with anti-AQP3 or anti-Nox2 showing the interaction between endogenous AQP3 and Nox2. Figure 5: AQP3-dependent H 2 O 2 permeability in keratinocytes. ( a , b ) H 2 O 2 uptake into primary cultured keratinocytes. Keratinocytes were incubated with H 2 O 2 (10 to 300 μM), and cellular H 2 O 2 was detected using CM-H 2 DCFDA fluorescence using a plate reader. ( a ) Representative fluorescence intensity of CM-H 2 DCFDA. ( b ) Increased fluorescence intensity at 15 s after addition of H 2 O 2 (s.e., n =5, * P <0.01, H 2 O 2 added versus control cells by t -test). ( c – d ) Intracellular H 2 O 2 was monitored by CM-H 2 DCFDA fluorescence with TNF-α stimulation (100 ng ml −1 ). ( c ) Representative fluorescence intensity in WT and AQP3 −/− cells. ( d ) Cells were incubated with DPI (5 μM), catalase (2,000 U ml −1 ) or vehicle (PBS) for 30 min, and followed by TNF-α (100 ng ml −1 ) for 30 s (s.e., n =5, * P <0.01 by t -test). ( e ) WT and AQP3 −/− cells transfected with HyPer were incubated with TNF-α (100 ng ml −1 ) or H 2 O 2 (100 μM) for 3 min. Representative immunofluorescence. Scale bar, 20 μm. ( f ) Cellular H 2 O 2 after stimulation by TNF-α (100 ng ml −1 ) or H 2 O 2 (100 μM) in primary keratinocytes from WT, AQP3 −/− , or Nox2 −/− mice using CM-H 2 DCFDA fluorescence (1 min, s.e., n =7, * P <0.01 by t -test). ( g ) Left: immunoblot of AQP3 and Nox2 in membrane-rich fraction from WT, AQP3 −/− and Nox2 −/− keratinocytes. Right: cell lysates by RIPA were immunoprecipitated with anti-AQP3 or anti-Nox2 showing the interaction between endogenous AQP3 and Nox2. Full size image Extracellular H 2 O 2 , which is mainly produced by the activation of plasma membrane NADPH oxidase (Nox) in response to various stimulation including TNF-α, is believed to be highly diffusible across the membrane and to act as a second messenger [17] , [18] , [30] , [40] , [41] . TNF-α stimulation markedly increased intracellular H 2 O 2 in WT mouse keratinocytes within 30 s ( Fig. 5c ). Pretreatment with diphenyleneiodonium (DPI), a general Nox inhibitor, or incubation with catalase, which removes any extracellular H 2 O 2 , greatly reduced the TNF-α-induced increase intracellular H 2 O 2 in WT cells, suggesting that TNF-α stimulation activates Nox for extracellular production of H 2 O 2 ( Fig. 5d ). The TNF-α-induced increase in intracellular H 2 O 2 level was remarkably reduced in AQP3 −/− keratinocytes, and neither DPI nor catalase treatment affected cellular H 2 O 2 ( Fig. 5d ). To verify the TNF-α-mediated increase in the intracellular H 2 O 2 by an independent method, cells were transfected with HyPer, a genetically encoded ratiometric sensor that is selective to H 2 O 2 and allows dynamic monitoring of intracellular H 2 O 2 concentration [42] . Confocal microscopy showed increased HyPer fluorescence in the cytosol and around the cell membrane after the addition of TNF-α (100 ng ml −1 ) or H 2 O 2 (100 μM) in WT cells, with much less fluorescence in AQP3 −/− cells ( Fig. 5e ). It was reported that human keratinocytes express both Nox1 and Nox2 (ref. 43 ). The involvement of Nox2 in TNF-α-mediated cellular H 2 O 2 induction was demonstrated using primary keratinocytes from Nox2 knockout (Nox2 −/− ) mice; Nox1 knockdown had little effect ( Supplementary Fig. 5c ). We found that the TNF-α-induced increase in intracellular H 2 O 2 level was suppressed in Nox2 −/− primary keratinocytes compared with WT cells, while the uptake of exogenous H 2 O 2 was not affected by Nox2 deficiency ( Fig. 5f ). These results indicated that extracellular H 2 O 2 produced by TNF-α stimulation is dependent on Nox2 in mouse keratinocytes. On the basis of the rapid increase in intracellular H 2 O 2 in response to TNF-α stimulation, we speculated that AQP3 may associate with Nox2 on the plasma membrane. Immunoprecipitation revealed an association between AQP3 and Nox2 in mouse primary keratinocytes ( Fig. 5g ). Together, these results support a model in which TNF-α stimulation induces extracellular H 2 O 2 production by Nox2 activation, which is rapidly transported intracellularly in keratinocytes through AQP3. AQP3-mediated cellular H 2 O 2 regulates NF-κB activation Next, we examined whether the intracellular H 2 O 2 level modulates TNF-α-induced NF-κB/p65 activation. Consistent with the immunoblot study in Fig. 4a , immunofluorescence showed that TNF-α stimulation translocated p65 into the nucleus in WT cells following NF-κB activation, with less translocation of p65 in AQP3 −/− cells ( Fig. 6a ). Treatment of WT cells with DPI or catalase suppressed TNF-α-induced p65 translocation into the nucleus, suggesting that the intracellular H 2 O 2 level modulates TNF-α-induced NF-κB/p65 activation ( Fig. 6a ). 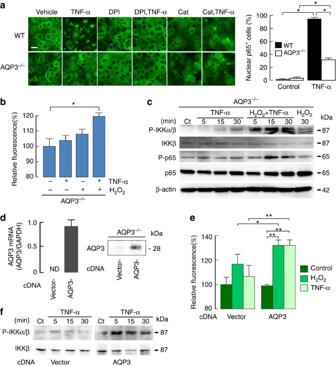Figure 6: AQP3-dependent H2O2accumulation in keratinocytes regulates NF-κB activation. (a) Left: representative immunofluorescence of p65 in keratinocytes from WT and AQP3−/−mice. Cells were stimulated with TNF-α (100 ng ml−1) for 1 h. Some cells were incubated with catalase (2,000 U ml−1) or DPI (5 μM) for 30 min before TNF-α stimulation. Scale bar, 20 μm. Right: numbers of p65 positive cells in the nucleus (s.e., over 100 cells from four different fields, *P<0.01 byt-test). (b,c) AQP3−/−primary keratinocytes were incubated with TNF-α (100 ng ml−1) and/or H2O2(300 μM). (b) Cellular H2O2level (1 min, s.e.,n=7, *P<0.01 byt-test). (c) Representative immunoblot with phospho-IKKα/β, IKKβ, phospho-p65, p65 and β-actin stimulated for indicated times. (d–f) AQP3−/−primary keratinocytes were transfected with mouse AQP3 cDNA or empty vector (pCMV6). (d) Left: mRNA analysed by quantitative RT–PCR. Right: immunoblotting with AQP3 antibody. (e) Cellular H2O2after stimulation with TNF-α (100 ng ml−1) or H2O2(100 μM; 1 min, s.e.,n=6, *P<0.05, **P<0.01 byt-test). (f) Immunoblot with phospho-IKKα/β or IKKβ stimulated with TNF-α (100 ng ml−1) for indicated times. Experiments incandfwere performed in two independent sets of experiments with similar results. Figure 6: AQP3-dependent H 2 O 2 accumulation in keratinocytes regulates NF-κB activation. ( a ) Left: representative immunofluorescence of p65 in keratinocytes from WT and AQP3 −/− mice. Cells were stimulated with TNF-α (100 ng ml −1 ) for 1 h. Some cells were incubated with catalase (2,000 U ml −1 ) or DPI (5 μM) for 30 min before TNF-α stimulation. Scale bar, 20 μm. Right: numbers of p65 positive cells in the nucleus (s.e., over 100 cells from four different fields, * P <0.01 by t -test). ( b , c ) AQP3 −/− primary keratinocytes were incubated with TNF-α (100 ng ml −1 ) and/or H 2 O 2 (300 μM). ( b ) Cellular H 2 O 2 level (1 min, s.e., n =7, * P <0.01 by t -test). ( c ) Representative immunoblot with phospho-IKKα/β, IKKβ, phospho-p65, p65 and β-actin stimulated for indicated times. ( d – f ) AQP3 −/− primary keratinocytes were transfected with mouse AQP3 cDNA or empty vector (pCMV6). ( d ) Left: mRNA analysed by quantitative RT–PCR. Right: immunoblotting with AQP3 antibody. ( e ) Cellular H 2 O 2 after stimulation with TNF-α (100 ng ml −1 ) or H 2 O 2 (100 μM; 1 min, s.e., n =6, * P <0.05, ** P <0.01 by t -test). ( f ) Immunoblot with phospho-IKKα/β or IKKβ stimulated with TNF-α (100 ng ml −1 ) for indicated times. Experiments in c and f were performed in two independent sets of experiments with similar results. Full size image Further studies were done to verify that AQP3-mediated H 2 O 2 transport regulates NF-κB activation. Because the addition of a high concentration of H 2 O 2 (over 300 μM) led to increase an intracellular H 2 O 2 level even in AQP3 −/− cells (shown in Fig. 5b ), AQP3 −/− cells were stimulated with TNF-α in the presence of 300 μM H 2 O 2 . TNF-α stimulation together with the addition of H 2 O 2 increased intracellular H 2 O 2 in AQP3 −/− cells, in which H 2 O 2 uptake probably occurs by passive diffusion across the plasma membrane ( Fig. 6b ). In this setting, both IKKβ and p65 were activated in AQP3 −/− keratinocytes, while addition of 300 μM H 2 O 2 alone had less effect ( Fig. 6c , Supplementary Fig. 7 ). We speculate that AQP3-mediated H 2 O 2 accumulation may increase TNF-α-induced NF-κB activation. Next, we determined whether forced expression of AQP3 by transfection with mouse AQP3 cDNA in AQP3 −/− cells could rescue TNF-α-induced NF-κB activation by increasing intracellular H 2 O 2 . AQP3 expression was seen in AQP3 −/− cells following AQP3 transfection ( Fig. 6d , Supplementary Fig. 7 ). Both H 2 O 2 transport and the TNF-α-induced H 2 O 2 level were restored in AQP3 −/− cells by forced expression of AQP3 ( Fig. 6e ). In this setting, TNF-α-induced IKKβ phosphorylation was increased compared with control (empty vector transfected) AQP3 −/− cells ( Fig. 6f , Supplementary Figs 6b and 7 ). Taken together, these results suggest that TNF-α-induced NF-κB cell signalling require a threshold concentration of intracellular H 2 O 2 involving AQP3-facilitated membrane transport. H 2 O 2 inactivates PP2A and regulates NF-κB activation We next sought to identify the targets of AQP3-mediated H 2 O 2 within the NF-κB pathway. Signalling with H 2 O 2 is believed to be mediated by oxidation of the critical cysteine residues of target proteins, including protein tyrosine phosphatases and many other H 2 O 2 effector molecules [17] , [44] . It was hypothesized that AQP3-mediated H 2 O 2 modulates protein phosphatase 2A (PP2A) to regulate NF-κB activation, as PP2A has been shown to be inactivated by H 2 O 2 in redox-sensitive cysteine residues, to interact with the IKK complex and p65, and to regulate NF-κB activation [45] , [46] , [47] , [48] , [49] , [50] , [51] . PP2A activity, quantified by PP2A inhibitor okadaic acid (OA)-sensitive phosphatase activity, was measured in primary culture keratinocytes after TNF-α or H 2 O 2 addition. 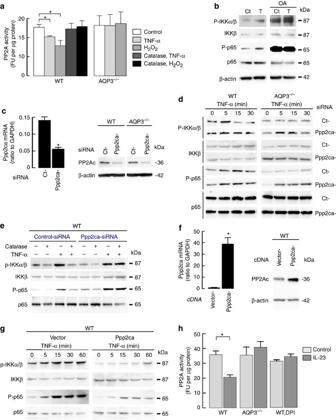Figure 7: TNF-α-mediated H2O2inactivates PP2A and regulates NF-κB activation. (a) PP2A activity in WT and AQP3−/−keratinocytes stimulated with TNF-α (100 ng ml−1) or H2O2(300 μM) for 10 min. Some cells were incubated with catalase (2,000 U ml−1) for 30 min before stimulation. PP2A activity was calculated from the rate of dephosphorylation of a radioactive substrate per minute per microgram protein in the presence and absence of okadaic acid (OA, 10 μM), an inhibitor of PP2A (s.e.,n=5, *P<0.01 byt-test). (b) WT keratinocytes were incubated with OA (10 μM, 30 min) and stimulated with TNF-α (100 ng ml−1, 15 min). Immunoblot with anti-phospho-IKKα/β, IKKβ, phospho-p65, p65 and β-actin. (c–e) Ppp2ca knockdown in WT and AQP3−/−keratinocytes by siRNA transfection. (c) PP2A expression by quantitative RT–PCR and immunoblotting (s.e.,n=4, *P<0.01 byt-test). (d) Cells were stimulated with TNF-α (100 ng ml−1). Representative immunoblot with phospho-IKKα/β, IKKβ, phospho-p65 and p65. (e) WT cells with control- or Ppp2ca-siRNA transfection were incubated with catalase (2,000 U ml−1, 30 min) before TNF-α stimulation. (f,g) WT keratinocytes were transfected with empty vector (pCMV6) or plasmid-expressing mouse Ppp2ca. (f) PP2A overexpression was analysed by quantitative RT–PCR and immunoblotting (s.e.,n=4, *P<0.01 byt-test). (g) Representative immunoblot of phospho-IKKα/β, IKKβ, phospho-p65 and p65 with TNF-α (100 ng ml−1) stimulation. (h) Mice were injected IL-23 into the ear as described inFig. 1and PP2A activity was measured in epidermal homogenates. Some WT mice were injected DPI (2 μg g−1weight) intravenously 1 h before IL-23 injection (s.e.,n=3–5, *P<0.01 byt-test). Experiments ind,eandgwere performed in two additional sets of independent experiments with similar results. Figure 7a shows reduced PP2A activity in response to H 2 O 2 or TNF-α addition in WT cells, while neither H 2 O 2 nor TNF-α affected PP2A activity in AQP3 −/− cells. Pretreatment of WT cells with catalase attenuated the decrease in PP2A activity in response to TNF-α or H 2 O 2 ( Fig. 7a ). These data indicate that the TNF-α-mediated increase in H 2 O 2 inactivates PP2A in WT but not AQP3 −/− cells. Figure 7: TNF-α-mediated H 2 O 2 inactivates PP2A and regulates NF-κB activation. ( a ) PP2A activity in WT and AQP3 −/− keratinocytes stimulated with TNF-α (100 ng ml −1 ) or H 2 O 2 (300 μM) for 10 min. Some cells were incubated with catalase (2,000 U ml −1 ) for 30 min before stimulation. PP2A activity was calculated from the rate of dephosphorylation of a radioactive substrate per minute per microgram protein in the presence and absence of okadaic acid (OA, 10 μM), an inhibitor of PP2A (s.e., n =5, * P <0.01 by t -test). ( b ) WT keratinocytes were incubated with OA (10 μM, 30 min) and stimulated with TNF-α (100 ng ml −1 , 15 min). Immunoblot with anti-phospho-IKKα/β, IKKβ, phospho-p65, p65 and β-actin. ( c – e ) Ppp2ca knockdown in WT and AQP3 −/− keratinocytes by siRNA transfection. ( c ) PP2A expression by quantitative RT–PCR and immunoblotting (s.e., n =4, * P <0.01 by t -test). ( d ) Cells were stimulated with TNF-α (100 ng ml −1 ). Representative immunoblot with phospho-IKKα/β, IKKβ, phospho-p65 and p65. ( e ) WT cells with control- or Ppp2ca-siRNA transfection were incubated with catalase (2,000 U ml −1 , 30 min) before TNF-α stimulation. ( f , g ) WT keratinocytes were transfected with empty vector (pCMV6) or plasmid-expressing mouse Ppp2ca. ( f ) PP2A overexpression was analysed by quantitative RT–PCR and immunoblotting (s.e., n =4, * P <0.01 by t -test). ( g ) Representative immunoblot of phospho-IKKα/β, IKKβ, phospho-p65 and p65 with TNF-α (100 ng ml −1 ) stimulation. ( h ) Mice were injected IL-23 into the ear as described in Fig. 1 and PP2A activity was measured in epidermal homogenates. Some WT mice were injected DPI (2 μg g −1 weight) intravenously 1 h before IL-23 injection (s.e., n =3–5, * P <0.01 by t -test). Experiments in d , e and g were performed in two additional sets of independent experiments with similar results. Full size image We next determined the effect of PP2A inhibition on TNF-α-induced NF-κB activation in WT keratinocytes. Figure 7b shows that OA treatment before TNF-α stimulation greatly enhanced phosphorylation of IKKβ and p65 even in the absence of TNF-α stimulation ( Supplementary Fig. 7 ). To further investigate the role of PP2A in TNF-α-induced NF-κB activation, we knocked down Ppp2ca, the catalytic subunit of PP2A, in WT and AQP3 −/− keratinocytes ( Fig. 7c , Supplementary Fig. 7 ). Ppp2ca knockdown of AQP3 −/− cells rescued the reduced TNF-α-induced NF-κB activation, including phosphorylation of IKKβ and p65 ( Fig. 7d , Supplementary Figs 6c and 7 ). Moreover, pretreatment with catalase suppressed the TNF-α-induced phosphorylation of IKKβ and p65 in WT cells, while Ppp2ca knockdown ameliorated the effect of catalase on WT cells ( Fig. 7e , Supplementary Fig. 7 ). As further evidence for the involvement of PP2A in TNF-α-NF-κB cell signalling, Ppp2ca was overexpressed in WT keratinocytes ( Fig. 7f , Supplementary Fig. 7 ) and NF-κB activation in response to TNF-α was analysed. Figure 7g shows that Ppp2ca overexpression suppressed TNF-α-induced phosphorylation of IKKβ and p65 ( Supplementary Figs 6d and 7 ). Last, we determined the effect of IL-23 application on PP2A activity in vivo . PP2A activity was significantly decreased in WT epidermal homogenates with IL-23 application compared with control, while PP2A activity was unaffected by IL-23 treatment in AQP3 −/− epidermis ( Fig. 7h ). The administration of low-dose DPI has been used to inhibit Nox in vivo [52] . DPI administration before IL-23 injection suppressed the decrease in PP2A activity, implying an effect of Nox-derived H 2 O 2 on PP2A activity in vivo . Collectively, these data suggest that PP2A is a target of AQP3-mediated H 2 O 2 elevation involved in NF-κB activation. TNF-α-induced NF-κB activation depends on AQP3 in NHEK The involvement of AQP3 in TNF-dependent NF-κB activation was studied using AQP3 knockdown in human primary keratinocytes (NHEK). Transfection of short interfering RNA (siRNA)-AQP3 into NHEK successfully reduced AQP3 mRNA and protein expression ( Fig. 8a , Supplementary Fig. 7 ). H 2 O 2 transport was decreased in AQP3 knockdown cells compared with control-siRNA transfected cells ( Fig. 8b ). The increase in intracellular H 2 O 2 following TNF-α was also reduced by AQP3 knockdown ( Fig. 8b ), as was TNF-α-induced NF-κB activation as shown by phosphorylation of IKKβ and p65 ( Fig. 8c , Supplementary Figs 6e and 7 ). Quantitative RT–PCR showed that TNF-α stimulation increased IL-17C and IL-6 transcript expression, with lesser increases in AQP3 knockdown keratinocytes ( Fig. 8d ). 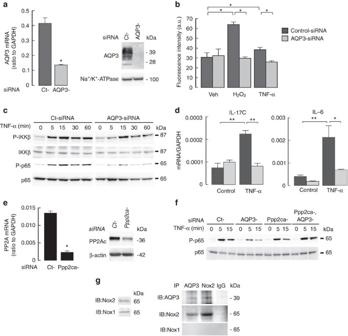Figure 8: TNF-α induced NF-κB activation depends on AQP3 in human primary keratinocytes. NHEK were transfected with AQP3 or non-targeting (Ct) siRNA. (a) Left: relative mRNA expression of AQP3/GAPDH (s.e.,n=4, *P<0.01 byt-test). Right: immunoblot of membrane fraction with anti-AQP3 and anti-Na+/K+-ATPase. (b) Cellular H2O2levels determined by CM-H2DCFDA after TNF-α (100 ng ml−1) or H2O2(10 μM) stimulation (30 s, s.e.,n=5, *P<0.01 byt-test). (c) Immunoblot with phospho-IKKβ, IKKβ, phospho-p65 and p65 after TNF-α stimulation. (d) mRNA expression of IL-17C and IL-6 by real-time RT–PCR. Cells were incubated with TNF-α (50 ng ml−1) for 24 h. Data are expressed as the ratio to GAPDH (s.e.,n=5, *P<0.05, **P<0.01 byt-test). (e) Ppp2ca knockdown in NHEK by siRNA transfection (s.e.,n=4, *P<0.01 byt-test). (f) Immunoblot with phospho-p65 and p65 after TNF-α stimulation in AQP3 and/or Ppp2ca knockdown cells. Experiments incandfwere performed in two additional sets of independent experiments with similar results. (g) NHEK cell lysates were immunoprecipitated with anti-AQP3 or anti-Nox2 antibodies, showing interaction between AQP3 and Nox2. Figure 8: TNF-α induced NF-κB activation depends on AQP3 in human primary keratinocytes. NHEK were transfected with AQP3 or non-targeting (Ct) siRNA. ( a ) Left: relative mRNA expression of AQP3/GAPDH (s.e., n =4, * P <0.01 by t -test). Right: immunoblot of membrane fraction with anti-AQP3 and anti-Na + /K + -ATPase. ( b ) Cellular H 2 O 2 levels determined by CM-H 2 DCFDA after TNF-α (100 ng ml −1 ) or H 2 O 2 (10 μM) stimulation (30 s, s.e., n =5, * P <0.01 by t -test). ( c ) Immunoblot with phospho-IKKβ, IKKβ, phospho-p65 and p65 after TNF-α stimulation. ( d ) mRNA expression of IL-17C and IL-6 by real-time RT–PCR. Cells were incubated with TNF-α (50 ng ml −1 ) for 24 h. Data are expressed as the ratio to GAPDH (s.e., n =5, * P <0.05, ** P <0.01 by t -test). ( e ) Ppp2ca knockdown in NHEK by siRNA transfection (s.e., n =4, * P <0.01 by t -test). ( f ) Immunoblot with phospho-p65 and p65 after TNF-α stimulation in AQP3 and/or Ppp2ca knockdown cells. Experiments in c and f were performed in two additional sets of independent experiments with similar results. ( g ) NHEK cell lysates were immunoprecipitated with anti-AQP3 or anti-Nox2 antibodies, showing interaction between AQP3 and Nox2. Full size image Last, we investigated the involvement of PP2A in AQP3-facilitated NF-κB activation in NHEK. Ppp2ca knockdown was done in control or AQP3 knockdown NHEK ( Fig. 8e , Supplementary Fig. 7 ). Ppp2ca knockdown restored the impaired TNF-α-induced p65 activation in AQP3 knockdown cells ( Fig. 8f , Supplementary Fig. 7 ). Again, reciprocal immunoprecipitation analysis showed association of AQP3 with Nox2 in NHEK ( Fig. 8g ). These results in human primary keratinocytes support the findings in mouse primary keratinocytes on the involvement of AQP3 in TNF-α-dependent H 2 O 2 induction and NF-κB signalling ( Fig. 9 ). 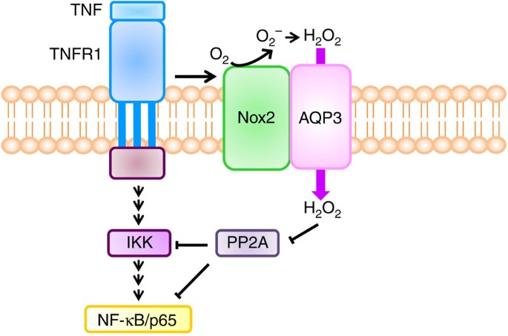Figure 9: Model of AQP3-mediated NF-κB activation. TNF-α binds to TNFR1 in keratinocytes and induces the production of H2O2by Nox2. Extracellular H2O2is rapidly transported intracellularly through AQP3. H2O2modifies PP2A, regulating IKKβ and/or NF-κB/p65 activation. Figure 9: Model of AQP3-mediated NF-κB activation. TNF-α binds to TNFR1 in keratinocytes and induces the production of H 2 O 2 by Nox2. Extracellular H 2 O 2 is rapidly transported intracellularly through AQP3. H 2 O 2 modifies PP2A, regulating IKKβ and/or NF-κB/p65 activation. Full size image We discovered here a novel role for AQP3 in the pathogenesis of psoriasis, which involved its H 2 O 2 transport function in keratinocytes. The uptake of extracellular H 2 O 2 by keratinocytes generated in response to TNF-α, which was required for NF-κB activation, was dependent on AQP3 as diagrammed in Fig. 9 . Keratinocytes made AQP3-deficient by gene knockout or knockdown showed reduced TNF-α-induced increase in intracellular H 2 O 2 and NF-κB activation. The reduced intracellular H 2 O 2 suppressed TNF-α-dependent NF-κB activation, while either exogenous H 2 O 2 supplementation or expression of AQP3 rescued the impaired NF-κB activation with restored intracellular H 2 O 2 levels in AQP3 −/− cells. In a mouse model of psoriasis produced by IL-23 application, there was continuous NF-κB activation and a higher H 2 O 2 concentration in keratinocytes of WT psoriatic skin, which was dependent on TNF-α signalling. AQP3 −/− mice showed remarkably impaired development of psoriasis, with reduced NF-κB activation and cellular H 2 O 2 . Together, these findings support the involvement of AQP3 in the development of psoriasis by a mechanism involving its H 2 O 2 transport function and downstream TNF-α-dependent NF-κB activation in keratinocytes. H 2 O 2 is emerging as a second messenger in cell signalling. Previous papers have proposed that the intracellular concentration of H 2 O 2 should rapidly exceed a certain threshold, probably 10–100 μM, to serve as a signalling molecule [30] , [53] , [54] . Extracellular H 2 O 2 produced by membrane Nox activation in response to receptor activation by ligands, such as growth factors, hormones and cytokines, has classically been thought to freely diffuse across biological membranes [17] , [55] . However, because H 2 O 2 is rapidly degraded in the cells by various enzymes, including catalase, glutathione peroxidases and peroxiredoxins [53] , [56] , continuous influx of H 2 O 2 may be necessary to elevate intracellular H 2 O 2 levels needed for cell signalling. Here, we found that TNF-α-induced production of extracellular H 2 O 2 was mainly dependent on Nox2 in keratinocytes, and that a membrane-associated AQP3–Nox2 complex may allow constitution of a localized signalling mechanism following TNF-α stimulation. AQP3 may thus be required to achieve a sufficiently high local concentration of H 2 O 2 near the membrane to act as a second messenger. H 2 O 2 has been implicated in the regulation of NF-κB; however, there is still no consensus on its role in NF-κB activation [30] , [57] . A recent study showed that dual oxidase 1-derived H 2 O 2 is involved in NF-κB signalling in skin in a zebrafish model [39] . Nevertheless, the molecular mechanism of NF-κB regulation by H 2 O 2 has been shown to be cell-type specific and to involve quite different mechanisms. There is evidence for cysteine residues being the most likely targets of Nox-mediated H 2 O 2 signalling [17] , [58] . Exposure to excess H 2 O 2 causes irreversible oxidation of the cysteine residues at the active sites of specific phosphatases such as PTEN and SHP1/2, resulting in their inhibition, which suppresses cell signalling [17] . The Ser/Thr phosphatases, including PP2A and PP1a, are also sensitive to H 2 O 2 modification, having H 2 O 2 -sensitive cysteine residues [59] . PP2A was reported to be inactivated by H 2 O 2 exposure or TNF-α stimulation [60] , [61] . Previous studies also indicated that PP2A-regulated NF-κB cell signalling involves modulation of IKK [45] , [46] , [47] , [48] , [51] , [62] . Consistent with these findings, a large-scale RNAi screen revealed that a PP2A catalytic or regulatory subunit associated IKK complex, p65, and/or Traf2, and led to the regulation of NF-κB [49] . Here, we showed that PP2A inactivation by H 2 O 2 exposure or TNF-α stimulation was dependent on AQP3 expression in WT primary keratinocytes. Ppp2ca knockdown in AQP3 −/− keratinocytes rescued the reduced IKKβ and p65 activation, while Ppp2ca knockdown in WT cells abrogated the effect of catalase on TNF-α-induced NF-κB activation. In contrast, Ppp2ca overexpression in WT keratinocytes suppressed IKKβ and p65 activation. Taken together, our data suggest that PP2A is one of the target proteins of AQP3-mediated H 2 O 2 uptake during TNF-α-induced NF-κB cell signalling, in which the increased H 2 O 2 may oxidize and inactivate PP2A through the cysteine residue and sequentially activate IKK and p65. Further studies are needed to establish the precise mechanism(s) linking PP2A with the regulation of TNF-α-induced NF-κB activation in keratinocytes. Regarding the redox state in psoriasis, there are increasing studies that showed higher levels of oxidative stress markers in psoriatic subjects, such as nitric oxide [63] , superoxide dismutase, catalase [64] , superoxide anions [65] and peroxiredoxin 2 (refs 66 , 67 ). A recent report also showed significantly higher H 2 O 2 and Nox activity in white blood cells of psoriatic patients compared with controls [68] . Although the activated redox state was proposed to cause DNA modification or inflammation, the underlying mechanisms involving redox state in the pathogenesis of psoriasis are not clear. Our findings suggest that keratinocyte-generated H 2 O 2 triggers psoriasis via modulation of NF-κB cell signalling, which clarifies the role of H 2 O 2 - and redox-mediated cell signalling in psoriasis. Previously, we reported impaired tumorigenesis in AQP3 −/− mice in a DMBA/PMA-induction model, but the underlying mechanism was unclear [13] . A number of studies support the involvement of ROS in cell growth, survival, metastasis and inflammation during cancer development and progression [69] . AQP3-mediated H 2 O 2 transport may provide an additional or alternative mechanism for the impaired skin tumorigenesis in AQP3 −/− mice. There is currently a controversy regarding the primary pathogenic functions of keratinocytes versus T cells in psoriasis [1] , [2] , [3] . The psoriasis model in this study uses IL-23, which may induce downstream signal molecules including TNF-α and IL-22 (refs 23 , 24 ). Our results suggested the requirement of AQP3 expression in both keratinocytes and T cells for the development of psoriasis induced by IL-23 application. We here identified a link between AQP3 expression and NF-κB cell signalling in keratinocytes that was associated with the development of psoriasis. Regarding the function of AQP3 in T cells, the current study together with our previous findings [16] suggest the involvement of AQP3 in T cell chemotaxis into the dermal and epidermal layer, a critical step for initiation of the immune response in the development of psoriasis. Further studies will determine the role of AQP3 in the crosstalk between keratinocytes and T cells in the pathogenesis of psoriasis. In summary, our data implicate a novel role of AQP3 in the pathogenesis of psoriasis in which AQP3-mediated intracellular H 2 O 2 uptake is required for TNF-α-induced NF-κB activation in epidermal keratinocytes. Our findings support AQP3 as a novel determinant in psoriasis and hence a potential new therapeutic target. Mice AQP3 −/− mice (C57BL/6 genetic background) were generated by targeted gene disruption [70] . Nox2 knockout mice (Nox2 −/− , gp91 phox - , C57BL/6 genetic background) were purchased from The Jackson Laboratory (Bar Harbor, MA). Eight- to 10-week-old female mice were used. All animal experiments were approved by the Committee on Animal Research of Kyoto University. Psoriasis-like mouse models IL-23 (500 ng in 40 μl PBS, Miltenyi Biotec) or vehicle control (PBS, 40 μl) was intradermally injected daily into the ear skin of WT and AQP3 −/− mice for 4 days [23] , [24] . Mice were killed at 24 h after the final IL-23 injection and skin samples were excised. Human subjects A total of 18 patients with psoriasis and five healthy volunteers were enrolled in this study. Informed consent was obtained from all the subjects. The study was approved by the Ethics Committee of the Kyoto University. Primary culture of mouse and human keratinocytes Full-thickness skin samples from 1-day-old mice were incubated in dispase II (5 U ml −1 ; Boehringer Mannheim) overnight at 4 °C. The epidermis was separated from the dermis, cut into fragments and incubated in 0.25% trypsin-0.1% EDTA for 10 min. Cells were seeded on collagen type I plates (BD Biosciences) and cultured in keratinocyte growth medium (Lonza) at 37 °C under 5% CO 2 . Neonatal human keratinocytes (NHEK, KK-4009, Kurabo, Japan) were grown in keratinocyte growth medium (Lonza) at 37 °C under 5% CO 2 . Cellular H 2 O 2 analysis Cellular H 2 O 2 was assayed using the CM-H2DCFDA reagent (Invitrogen) according to the manufacturer’s instructions using flow cytometry (FACS Fortessa system, Becton Dickinson, San Diego, CA) or a microplate reader (Flex station, Molecular Devices; or Envision, PerkinElmer Life Sciences). To monitor cellular H 2 O 2 in the skin, mice were injected with H 2 DCFDA intravenously (10 nmol g −1 , Invitrogen) 1 h before being killed. Cellular H 2 O 2 was observed in frozen section by fluorescence microscopy. To quantify cellular H 2 O 2 in mouse skin by FACS analysis, the excised skin was trypsinized and single epidermal cells were incubated with H 2 DCFDA. Immunoblotting and immunoprecipitation Cells were lysed with RIPA buffer (Cell Signaling Technology) for cell signalling analysis or with membrane extraction buffer (HEPES pH 7.4, 250 mM sucrose, 1 mM EDTA, 1 mM EGTA, 1% protease inhibitor cocktail) for membrane protein analysis. The supernatant (10,000 g , 10 min, 4 °C) was used for immunoblotting with antibodies against phospho-p65, p65, phospho-IKKβ, IKKβ, phosphor-Iκβα, Iκβα (Cell Signaling, 1:1,000), phospho- IKKα/β (Abcam, 1:500), AQP3 (Millipore, 1:1,000), Nox2 (Santa Cruz, 1:200 or Millipore, 1:1,000), PP2A or β-actin (Sigma, 1:2,000). For immunoprecipitation, protein lysate in RIPA was incubated with anti-TNF receptor I (R&D system, 1 μg antibody per 200 μg total protein), anti-AQP3 (Santa Cruz, 2 μg antibody per 400 μg total protein) or anti-Nox2 (Santa Cruz, 2 μg antibody per 400 μg total protein), and protein A or G agarose beads (GE Healthcare) at 4 °C overnight. Immunoblots were performed with anti-Traf2, RIP1 (Cell Signaling, 1:1,000), TNFR1 (R&D system, 1:1,000), AQP3 (Millipore, 1:1,000), Nox2 (Santa Cruz, 1:200 or Millipore, 1:1,000) or Nox1 (Millipore, 1:1,000). The horseradish peroxidase-conjugated secondary anti-rabbit or anti-mouse IgG antibody (Cell Signaling Technology, 1:1,000) were used and visualized by chemiluminescence (GE Healthcare). The optical density of the bands was quantified using Image J (National Institutes of Health, Supplementary Fig. 6 ). PP2A assay PP2A activity was assessed in primary keratinocytes using ProFluor Ser/Thr PPase assay kit (Promega) according to the manufacturer’s instructions. RNAi and plasmid DNAs Cells were transfected using Lipofectamine 2000 (Invitrogen) with Ppp2ca-, AQP3- or non-targeting-siRNA (ON-TARGET plus SMART pool, Thermo Scientific). The cDNA plasmids for AQP3, Ppp2ca (pCMV6 vector, Origine) or Hyper (pHyPer-cyto vector, Evrogen) was also transfected with Lipofectamine 2000. Using these methods, we generally found that 65–80% cells become positive after transfection. Immunofluorescence and immunohistochemistry For p65 immunofluorescence, cells were fixed with 4% formalin and permeabilized with 0.1% Triton X-100 and immunostained with p65 (Cell Signaling, 1:100) and anti-rabbit secondary antibody (FITC, Sigma, 1:200). Paraffin-embedded sections were stained with haematoxylin and eosin, anti-phospho-p65 antibody (Cell Signaling, 1:200) or Ki67 (Cell Signaling, 1:100). Bone marrow transplantation For bone marrow (BM) transplantation, red blood cells from WT and AQP3 −/− mice were subjected to hypotonic cell lysis. WT and AQP3 −/− recipients (8–10 weeks old) were γ-irradiated with two doses of 600 rad, 3 h apart. After irradiation, the mice received 10 6 BM cells intravenously. This protocol consistently gave >95% reconstitution of the recipient by donor haematopoietic cells, as evaluated by separate transplantation experiments using BM from C57BL/6-CD45.1 congenic mice ( Supplementary Fig. 2a ). The psoriasis mouse model was performed 2 months later. RNA extraction and real-time quantitative RT–PCR Total RNA was extracted using TRIZOL (Invitrogen). The cDNA was reverse transcribed from total RNA using the Prime Script RT reagent kit (Takara Bio, Otsu, Japan). Quantitative RT–PCR was performed using SYBR Green I (Takara Bio) and the Light Cycler real-time PCR apparatus (Roche). Primer sequences are listed in Supplementary Table 1 . Statistical analysis Statistical analysis was performed using the two-tailed Student’s t -test or analysis of variance. How to cite this article: Hara-Chikuma, M. et al. Aquaporin-3-mediated hydrogen peroxide transport is required for NF-κB signalling in keratinocytes and development of psoriasis. Nat. Commun . 6:7454 doi: 10.1038/ncomms8454 (2015).